Neuroligin-associated microRNA-932 targets actin and regulates memory in the honeybee Increasing evidence suggests small non-coding RNAs (ncRNAs) such as microRNAs (miRNAs) control levels of mRNA expression during experience-related remodelling of the brain. Here we use an associative olfactory learning paradigm in the honeybee Apis mellifera to examine gene expression changes in the brain during memory formation. Brain transcriptome analysis reveals a general downregulation of protein-coding genes, including asparagine synthetase and actin, and upregulation of ncRNAs. miRNA–mRNA network predictions together with PCR validation suggest miRNAs including miR-210 and miR-932 target the downregulated protein-coding genes. Feeding cholesterol-conjugated antisense RNA to bees results in the inhibition of miR-210 and of miR-932. Loss of miR-932 impairs long-term memory formation, but not memory acquisition. Functional analyses show that miR-932 interacts with Act5C , providing evidence for direct regulation of actin expression by an miRNA. An activity-dependent increase in miR-932 expression may therefore control actin-related plasticity mechanisms and affect memory formation in the brain. Non-coding RNAs (ncRNAs) including microRNAs (miRNAs) regulate gene expression at all known levels of cell development including the nervous system [1] , [2] , [3] . These molecules function by repressing gene expression at the post-transcriptional level through binding, usually at the 3′-untranslated region (3′UTR) of a target mRNA, thereby providing a dynamic brake on protein synthesis [4] . Recent studies suggest that combinations of miRNAs have been preconfigured through evolution to regulate groups of molecules that function in the same process, such as cell remodelling or synaptic development processes that underpin learning and memory [5] , [6] , [7] , [8] . This is supported by the number of overrepresented miRNA-target sites found in the 3′UTRs of mRNAs that make up functional pathways of the nervous system [9] . Although miRNA regulation of neuronal plasticity is thought to be a conserved mechanism among higher eukaryotes, there are few vertebrate and even fewer invertebrate studies that have attempted to characterize the specific roles of miRNAs in learning and memory [7] , [8] , [10] . The use of tractable insect models such as the honeybee that offers a sophisticated behavioural repertoire, a complete genome sequence, emerging RNA interference technologies and demonstrated adult brain plasticity provides an excellent opportunity to study molecular mechanisms underlying learning and memory [11] . Structural and functional plasticity of the honeybee brain has been extensively studied with respect to many different learning and memory paradigms. Olfactory learning of floral scents is an essential part of the honeybee’s foraging biology, and it has thus been particularly well investigated. Most studies use the proboscis extension response (PER) assay, which is an olfactory-conditioning assay, where bees learn to associate an odour with a food reward [12] . In honeybees odour learning and memory has been shown to consist of distinctive phases: short-term memory, mid-term memory and long-term memory (LTM) [13] , [14] , [15] , equivalent to what has been described for vertebrates. Each phase depends on different molecular pathways with LTM requiring ~10 h to form and notably depending on translational (early stage) and also transcriptional (late stage) processes [6] , [16] . This knowledge provides an important framework to examine the role of miRNAs in regulating different classes of memory. Here we examine molecular changes associated with LTM including upregulation of miRNAs and their downregulated target mRNAs that are putatively involved in the development and management of memory circuits arising from the learning of sensory cues. It has previously been reported that miR-932 is nested within intron 2 of the neuroligin 2 ( Nlg2 ) gene in the bee [17] . Although the neuroligins are highly conserved and have been shown to be involved in the development of glutamatergic and GABAergic synapses in vertebrates and invertebrates [17] , [18] , [19] , miR-932 is only conserved in insects. We show that miR-932 modulates LTM recall, but not memory acquisition. We also provide evidence how miRNAs work to control brain gene expression targeting cellular components such as the cytoskeleton, showing miR-932 directly targets actin and therefore regulates neuronal plasticity mechanisms associated with memory formation. Brain gene expression after olfactory learning and memory We used the PER assay to train honeybees to associate an odour with a sugar reward. Three groups of 60 foragers each were conditioned using 12 trials over 2 days, with six trials per day. Group one was conditioned with a mixture of 14 common floral odorants (floral mix) [20] , group two with the floral odour linalool and group three was exposed to air (no odour learning), thereby serving as baseline control. This procedure provided a focused olfactory learning experience for the bees of the first two groups, and ensured formation of a robust LTM. Bees from the conditioned groups learnt their respective odours well; there was no difference in performance between the groups conditioned to floral mix and conditioned to linalool (general linear model (GLM), F (1,1438) =0.251, P =0.107) ( Supplementary Fig. 1 ). By the second trial, group one showed 86.7% correct response to the floral mix, and group two showed 81.8% correct response to linalool. Both groups maintained this high level of learning (85–100% correct response) throughout the 2 days of conditioning until the last trial. The control group that was exposed to air showed no response, as no odour learning occurred in this group (significant difference to odour-conditioned groups: GLM, F (2,2157) =351.03, P <0.001). Immediately after completion of the olfactory conditioning, the brains of the bees from each group were dissected and RNA extracted for microarray analysis of gene expression. We found a total of 77 differentially expressed genes (DEGs) in the odour-conditioned groups (floral mix and linalool) compared with the control group (air) ( Supplementary Data 1 ). Although the first group was trained to a composite floral mix (14 odours) and the second only to a single odorant (linalool), the differential gene expression profile was very similar between the two groups (Pearson’s correlation=0.92; t =20.05; df=75; P <0.01). Most of the differentially expressed protein-coding genes (45 genes) of odour-conditioned bees were downregulated compared with the air group, with only 19% of the protein-coding genes (11 genes) upregulated ( Supplementary Data 1 ). Interestingly, 20 ncRNAs were found to be upregulated in both odour-conditioned groups (floral mix and linalool) and only one ncRNA was downregulated ( Supplementary Data 1 ). This suggests that ncRNAs might have an important role in the molecular regulation of olfactory learning and memory in honeybees. To validate the results obtained in the microarray transcriptome analysis, we investigated the expression levels of 23 DEGs by quantitative reverse transcription PCR (qRT-PCR) using the same RNA samples as for the microarrays. This analysis confirmed there was a significant positive correlation for both the floral mix (Pearson’s correlation=0.91; t =10.07; df=21; P <0.01) and linalool (Pearson’s correlation=0.88; t =8.37; df=21; P <0.01) ( Fig. 1 ). There was no significant difference between the two odour-conditioned groups, confirming that conditioning with either floral mix or linalool promotes similar changes in overall gene expression in the honeybee brain. 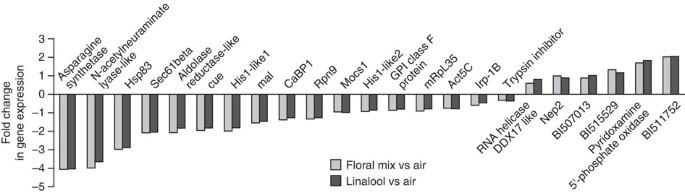Figure 1: qRT-PCR validation of 23 genes found differentially expressed in the microarray data from honeybee brains after olfactory conditioning. Honeybees were trained for 2 days with either a mixture of 14 floral odorants (floral mix) or single odour (linalool). The bars indicate the log2-change in gene expression normalized to RPL8 and compared with control bees (exposed only to air). Expression levels shown are means of three technical replicates for each sample. Figure 1: qRT-PCR validation of 23 genes found differentially expressed in the microarray data from honeybee brains after olfactory conditioning. Honeybees were trained for 2 days with either a mixture of 14 floral odorants (floral mix) or single odour (linalool). The bars indicate the log2-change in gene expression normalized to RPL8 and compared with control bees (exposed only to air). Expression levels shown are means of three technical replicates for each sample. Full size image Computational analysis of the protein–protein network To gain a global picture of the learning-induced DEGs we used a molecular systems approach. We constructed a putative protein–protein interaction (PPI) network for the genes that were differentially expressed in the odour-conditioned bees and their first-degree-interacting proteins ( Fig. 2 ; Supplementary Data 2 ). First, we used PPI data [21] to identify orthologous Drosophila fly genes and found that over 76% of the encoded proteins are also highly conserved in the honeybee genome (338 proteins and 441 PPIs). Most of the DEGs identified in odour-conditioned bees appear to function in overlapping molecular pathways ( Table 1 ). We measured three basic structural properties of these complex networks, the average degree (number of neighbours), the network density (normalized average degree) and the average path length (degree of separation). We used these properties to assess whether the olfactory-conditioning PPI network was significantly different from PPI networks constructed from an equivalent number of randomly selected genes ( Fig. 2a,b ). We found that genes in the olfactory-conditioning PPI network were significantly more interconnected than expected by chance (Kolmogorov–Smirnov tests are shown in Fig. 2b ). 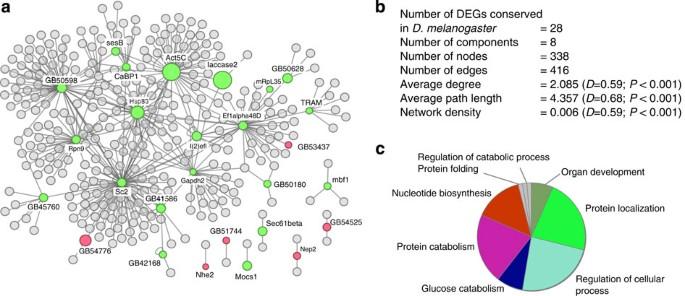Figure 2: Protein–protein interaction network and functional profile of DEGs associated with olfactory learning and memory. (a) PPI network of genes highly conserved in honeybee andDrosophilafly. Nodes represent proteins (Supplementary Data 2) shown with name or accession number (Beebase or Flybase). Edges depict interactions between proteins. Green nodes represent downregulated and red nodes upregulated genes in the microarray analysis of odour-conditioned bees. The node size is proportional to their level of differential expression (Supplementary Data 1). (b) The structural properties of the PPI network are significantly different from those expected by chance. The Kolmogorov–Smirnov tests for average degree, average path length and network density are shown in brackets. (c) Functional analysis showing significantly enriched Gene Ontology terms for those genes in the PPI network. Figure 2: Protein–protein interaction network and functional profile of DEGs associated with olfactory learning and memory. ( a ) PPI network of genes highly conserved in honeybee and Drosophila fly. Nodes represent proteins ( Supplementary Data 2 ) shown with name or accession number (Beebase or Flybase). Edges depict interactions between proteins. Green nodes represent downregulated and red nodes upregulated genes in the microarray analysis of odour-conditioned bees. The node size is proportional to their level of differential expression ( Supplementary Data 1 ). ( b ) The structural properties of the PPI network are significantly different from those expected by chance. The Kolmogorov–Smirnov tests for average degree, average path length and network density are shown in brackets. ( c ) Functional analysis showing significantly enriched Gene Ontology terms for those genes in the PPI network. Full size image Table 1 Functional enrichment analysis of differentially expressed genes in brains of honeybees after olfactory conditioning. Full size table The main hubs in the PPI network represent proteins encoded by genes, which were downregulated in odour-conditioned bees. These genes are known to be involved in the cytoskeleton organization ( Act5C and Hsp83 ), lipid metabolic process ( Sc2 ) and glucose catabolic process ( Gapdh2 , GB50598). Other important functional hubs comprised genes associated with protein localization ( Act5C , Sec61beta , TRAM and GB41586), regulation of cellular processes ( l(2)efl , Hsp83 , Rpn9 , Sec61beta , mbf1 , CaBP1 and GB54525), regulation of catabolic processes ( l(2)efl and Sec61beta ), protein folding ( Hsp83 ) and organ development ( Act5C , Hsp83 , sesB ) ( Fig. 2c ; Supplementary Data 3 ). We note enzymes such as asparagine synthetase, N -acetylneuraminate lyase and aldolase reductase do not feature in the PPI network, because they are involved in the biosynthesis and catalysis of simple organic substrates such as amino acids and sugars. Nevertheless, they also form an important functional hub of the PER-conditioning experiment. Computational analysis of the miRNA-target network To test whether the 45 downregulated genes in odour-conditioned bees were potentially dysregulated by miRNAs, we constructed a putative miRNA-target network for A. mellifera . The miRNA regulatory elements (MREs) were predicted using only mature miRNA sequences described in the miFam (family classification information for homologous miRNA hairpin sequences) feature of the miRBase database [22] . The mature miRNA sequences ( Supplementary Data 4 ) were used to identify putative miRNA-target sites in the 3′UTR of the 45 downregulated genes found in odour-conditioned bees. To reduce spurious hits, we compared miRNA-target sites in the 3′UTR of orthologous Drosophila genes, and only the consensus predictions found in both the bee and the fly were used to build the miRNA-target network ( Supplementary Data 5 ). The miRNA-target network was represented as a bipartite network where miRNAs are connected to target genes. The conserved miRNA-target network was composed of 28 target genes (62% of downregulated genes in the PER-conditioning experiment) and 64 miRNAs, with a total of 327 miRNA-target sites predicted from the 28 mRNA transcripts ( Supplementary Data 5 ). The average number of miRNA-target sites per gene is 11.7; of particular interest was Act5C , which seems to be targeted by 41 different miRNAs ( Supplementary Data 6 ). Other downregulated genes putatively targeted by >20 miRNAs include Ef1apha48D , cue , GB50180, asparagine synthetase and Mocs1 . We selected seven highly connected miRNAs (miR-34, miR-124, miR-210, miR-275, miR-278, miR-928 and miR-932) ( Supplementary Data 6 ) to evaluate their expression profile in the odour-conditioned bees, and performed qRT-PCR analyses using the same RNA samples as used for the microarray study. This revealed that all the selected miRNAs were upregulated in odour-conditioned bees albeit the floral mix-conditioned bees showed a more general increase in the level of miRNA expression compared with linalool-conditioned bees ( Fig. 3a ). To examine this relationship further, we constructed a composite miRNA–PPI network that was conserved between the honeybee and Drosophila ( Fig. 3b ). We again observed that Act5C ( actin ) is a major molecular hub that connects most of the predicted interactions within our network ( Figs 2a and 3b ). We chose two miRNAs, miR-210 and miR-932, to functionally validate our computational predictions based on their unique functions, genomic organization and levels of conservation; miR-932 is conserved in insects while miR-210 is highly conserved in all metazoa. A computational analysis of miRNAs in the honeybee genome showed that miR-932 is nested in the second intron of the Nlg2 gene putatively involved in synapse development [17] , [18] , [23] . In comparison, miR-210 is an independent RNA gene that functions in hypoxia response including targeting the Ephrin-A3 receptor in the nervous system [24] , [25] . miR-210 is also noted to be differentially expressed in bees performing different behavioural tasks such as brood care and foraging [26] . These miRNAs also have different targeting specificities: we predict miR-210 has 14 targets, whereas miR-932 only targets five DEGs found in the PER-conditioning experiment. When we consider predicted miRNA–mRNA interactions associated with the core PPI network ( Fig. 2a ), there were eight and four mRNA targets for miR-210 and miR-932, respectively ( Fig. 3b ). 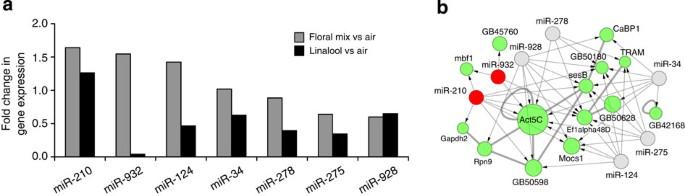Figure 3: Upregulated miRNAs in the odour-conditioned bees and the predicted mRNA–miRNA-target network. (a) qRT-PCR validation of seven miRNAs upregulated in odour-conditioned bees represented as a fold change in gene expression compared with the control group (air) using 18S rRNA as an endogenous control gene. Expression levels shown are means of three technical replicates for each sample. (b) Composite miRNA and PPI network conserved in honeybee and fruit fly. Green nodes represent target genes downregulated in odour-conditioned bees, and grey nodes represent selected miRNAs upregulated in odour-conditioned bees including miR-210 and miR-932 (red nodes) that we functionally characterized. Node labels are gene name or accession number (Beebase, Flybase and miRBase). Thick edges depict interactions between proteins and arrows depict predicted miRNA-binding sites. The size of the green nodes is proportional to their level of differential expression (Supplementary Data 1). Figure 3: Upregulated miRNAs in the odour-conditioned bees and the predicted mRNA–miRNA-target network. ( a ) qRT-PCR validation of seven miRNAs upregulated in odour-conditioned bees represented as a fold change in gene expression compared with the control group (air) using 18S rRNA as an endogenous control gene. Expression levels shown are means of three technical replicates for each sample. ( b ) Composite miRNA and PPI network conserved in honeybee and fruit fly. Green nodes represent target genes downregulated in odour-conditioned bees, and grey nodes represent selected miRNAs upregulated in odour-conditioned bees including miR-210 and miR-932 (red nodes) that we functionally characterized. Node labels are gene name or accession number (Beebase, Flybase and miRBase). Thick edges depict interactions between proteins and arrows depict predicted miRNA-binding sites. The size of the green nodes is proportional to their level of differential expression ( Supplementary Data 1 ). Full size image miR-932 and miR-210 are expressed in higher brain centres To determine the localization of miR-932 and miR-210 we performed in situ hybridizations of adult honeybee brains using LNA (locked nucleic acid) miRNA probes (Exiqon) to detect their RNA transcripts. Both miRNAs were predominantly expressed in the Kenyon cells of the mushroom bodies and to a lesser extent the cells surrounding the antennal lobes ( Fig. 4a,b,d ). Some differential staining was observed, with the miR-932 probe staining cell layers between the medulla and lobula regions of the visual system ( Fig. 4c ), and the central complex including weak punctate staining of protocerebrum and lateral horn. The scrambled control probe produced no staining ( Fig. 4e ). The mushroom bodies are higher-order brain centres responsible for the majority of the sensory integration and memory formation in the honeybee [13] , [14] , [27] . We found that the localization of miR-932 was similar to that of a number of molecules that function in synaptic development, including Nlg3 and neurexin 1 ( Nrx1 ) [17] albeit RNA transcripts of synaptic molecules are more generally expected to be associated with the majority of cell bodies in the honeybee brain. Considering the nested organization of Nlg2 and miR-932, we expected their expression to be highly correlated. However, Nlg2 and miR-932 expression seem to be discordant as Nlg2 is not significantly upregulated during olfactory learning [23] . Recent studies suggest there is a poor relationship between miRNA and host gene expression [28] , [29] , ~35% of intronic miRNAs are predicted to have their own promoter elements including regulatory sites for RNA polymerase II or III [30] , [31] . Bioinformatics analyses identified putative polymerase III A-box (5′-TAGCAGAATTGG-3′) and B-box (5′-GGTGTCGAAAC-3′) regulatory sites within 7 kb upstream of miR-932, suggesting this miRNA may be independently regulated. We similarly found a highly conserved B-box sequence (5′-GGCGTCGAACC-3′) 9 kb upstream of the miR-210. 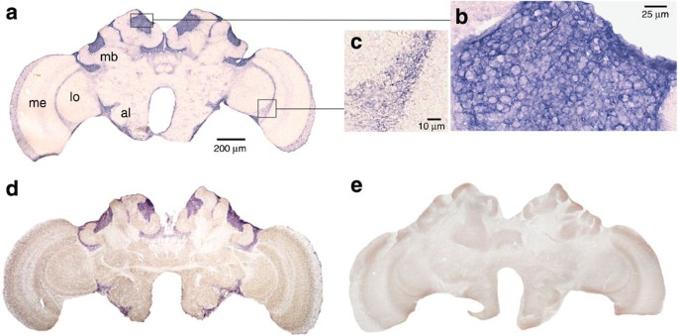Figure 4:In situRNA hybridization of 20-μm cross-sections of a forager honeybee brain, showing staining of miR-932 (a) and miR-210 (d). Both miR-932 and miR-210 are highly transcribed (magenta colour) in the Kenyon cells of the mushroom bodies (mb), see inset (b), and in cells surrounding the antennal lobes (al). Some differential staining of miR-932 is seen in cell layers between the medulla (me) and lobula (lo), see inset (c). A scrambled control probe showed no specific staining (e). Figure 4: In situ RNA hybridization of 20-μm cross-sections of a forager honeybee brain, showing staining of miR-932 (a) and miR-210 (d). Both miR-932 and miR-210 are highly transcribed (magenta colour) in the Kenyon cells of the mushroom bodies (mb), see inset ( b ), and in cells surrounding the antennal lobes (al). Some differential staining of miR-932 is seen in cell layers between the medulla (me) and lobula (lo), see inset ( c ). A scrambled control probe showed no specific staining ( e ). Full size image Function of miR-932 and miR-210 in learning and memory To determine whether miR-932 and miR-210 indeed play a regulatory role in learning and memory, we measured odour learning and memory recall in bees that were treated with miRNA inhibitors (antagomirs). Treatment was non-invasive: bees were fed cholesterol-conjugated antagomirs (antisense miRNA sequences, 1 μg antagomir diluted in 1 μl sugar solution) designed to specifically inhibit mature miR-932 and miR-210. Four treatment groups of at least 30 bees each were compared: sugar (behavioural control), scrambled control (nonsense RNA nucleotide sequence), antagomir-932 (a-miR-932) and antagomir-210 (a-miR-210). Twenty-four hours after treatment, bees were conditioned to a single odour (linalool) using the PER assay ( Fig. 5a ). The results showed that there was a significant main effect of trial during the training phase (GLM, F (5,859) =40.255, P <0.001), but no significant main effect of treatment (GLM, F (3,860) =1.375, P= 0.059), and no significant interaction between trial and treatment, (GLM, F (15,856) =0.123, P= 0.874). That is, all bees learnt the odour, and learning performance was equally good for all groups irrespective of treatment ( Fig. 5a ). A further 24 h after completion of odour conditioning, that is 48 h after treatment, all bees were assessed for LTM recall in the PER assay. On the basis of the current understanding of memory phases in honeybees, recall 24 h after conditioning relates to early LTM , which is translation dependent [15] , [32] . We found a significant main effect of treatment, (GLM, F (3,140) =5.302, P <0.001). Both control groups (sugar and scrambled) showed robust memory recall ( Fig. 5b ) with no significant difference between the controls (GLM, P =0.506). However, treatment with a-miR-932 resulted in significantly impaired memory recall compared with the sugar group (GLM, P <0.001), and the scrambled group ( P< 0.001). Treatment with a-miR-210 also reduced memory performance compared with the controls, but the statistical difference was only marginal (GLM, P =0.055 for sugar, P =0.049 for scrambled). Similarly, statistical difference compared with the a-miR-932-treated group was weak (GLM, P =0.042). 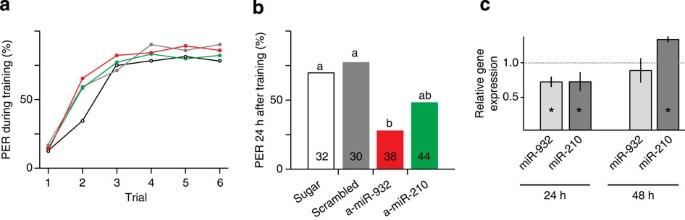Figure 5: Functional roles of miR-932 and miR-210 in learning and memory. (a) Learning curves for six odour-conditioning trials with linalool, showing percentage of correct proboscis extension response (PER), comparing bees 24 h after treatment with either sugar (white,n=32), scrambled antisense miRNA (grey,n=30), antisense miR-932 antagomir (red,n=38) or antisense miR-210 antagomir (green,n=44). (b) Memory recall in same groups of bees 48 h after treatment, showing percentage of correct PER; numbers in bars are numbers of bees per groups; different letters above bars indicate significant difference atP<0.05 (GLM). (c) Relative expression of miR-932 (light grey) and miR-210 (dark grey) in bee brains determined with qRT-PCR, 24 and 48 h after treatment with a-miR-932 and a-miR-210, respectively, compared with expression in brains treated with scrambled antisense miRNA as control. Sugar treatment was used as a calibrator group for calculating ΔΔCT. Expression levels shown are means±s.d. of three biological replicates compared with scrambled as baseline (dashed line). Statistical analysis was performed using Welch’st-test (*P<0.01). Figure 5: Functional roles of miR-932 and miR-210 in learning and memory. ( a ) Learning curves for six odour-conditioning trials with linalool, showing percentage of correct proboscis extension response (PER), comparing bees 24 h after treatment with either sugar (white, n =32), scrambled antisense miRNA (grey, n =30), antisense miR-932 antagomir (red, n =38) or antisense miR-210 antagomir (green, n =44). ( b ) Memory recall in same groups of bees 48 h after treatment, showing percentage of correct PER; numbers in bars are numbers of bees per groups; different letters above bars indicate significant difference at P <0.05 (GLM). ( c ) Relative expression of miR-932 (light grey) and miR-210 (dark grey) in bee brains determined with qRT-PCR, 24 and 48 h after treatment with a-miR-932 and a-miR-210, respectively, compared with expression in brains treated with scrambled antisense miRNA as control. Sugar treatment was used as a calibrator group for calculating ΔΔCT. Expression levels shown are means±s.d. of three biological replicates compared with scrambled as baseline (dashed line). Statistical analysis was performed using Welch’s t -test (* P <0.01). Full size image To validate the inhibition of memory recall by cholesterol antagomirs, we quantified miR-932 and miR-210 expression in bee brains using qRT-PCR. We showed there was a significant downregulation of miR-932 and miR-210 24 h after treatment with a-miR-932 and a-miR-210, respectively ( Fig. 5c ). Transcript levels of both miR-932 and miR-210 were significantly decreased by 30% (Welch’s t -test, P< 0.01). Forty-eight hours after antagomir treatment, the expression of miR-932 had almost recovered to baseline level, and expression levels of miR-210 were even higher than the baseline control (Welch’s t -test, P< 0.01) ( Fig. 5c ). It is not clear whether the return to baseline levels of the miRNAs 48 h after treatment is due to degradation of the antagomir and/or compensatory mechanisms that increase its endogenous expression. These results demonstrate that the non-invasive treatment of feeding antagomirs effectively inhibits miRNAs in the brain in a transient manner. As miR-210 only showed a marginal effect on LTM formation, we did not proceed with further experimental validation of this miRNA. Validation of miR-932 target genes We selected three genes that miR-932 putatively targets ( Act5C , Sec61b and His1 ) for functional analysis. These genes have functions that potentially affect learning and memory and activity-dependent neuronal plasticity such as cytoskeleton organization ( Act5C ), protein transportation ( Sec61b ) and chromatin organization ( His1 ). To examine the functional interaction of miR-932 and gene transcripts we used a pull-down assay and luciferase reporter system. Only predicted 3′UTR miRNA regulatory elements (MREs) with minimum free-energy hybridization score <−20 were considered for these analyses ( Supplementary Fig. 2 ). Although the coding regions of these three genes are highly conserved in insects, only Act5C has a miR-932 regulatory element (RE) that is conserved between honeybee and Drosophila. There are no Sec61b or His1 miR-932 REs that are conserved. To test potential Drosophila miR-932 target interactions we pulled down miRNA–mRNA complexes from Drosophila S2 cell lysates using a biotinylated miR-932 (bi-miR-932) probe and a biotinylated scrambled control (bi-scr) probe. We found Act5C transcripts were 10-fold enriched in RNA pulled down by bi-miR-932 compared with the bi-scr control. In comparison, there was only a small 1.5-fold enrichment of Sec61b and His1 transcripts in the RNA pull-down ( Supplementary Fig. 3 ). This suggests that Drosophila has a functional RE in the 3′UTR of Act5C that interacts with miR-932, confirming the miRNA-target predictions ( Fig. 3b ). To show orthologous honeybee transcripts with functional MREs are expressed in the brain, we RT-PCR amplified all three 3′UTR fragments that contained predicted miR-932 REs in Act5C , Sec61b and His1 from total mRNA extracted from the brains of forager bees ( Supplementary Fig. 2 ). To test whether the specific interactions of miR-932 with Act5C 3′UTR and its MREs found within this region can promote degradation of the Act5C mRNA, we used a luciferase reporter system to examine changes in expression of chimeric luciferase constructs mediated by miR-932 oligonucleotide mimics in vertebrate COS-7 cells. We used the psiCHECK2 (Ψ) system (Promega), which encodes two reporter genes: (1) the firefly ( Photinus pyralis ) luciferase (Fluc), and (2) the Renilla reniformis luciferase (Rluc) that contains a multiple cloning site for insertion of 3′UTRs or MREs from target analysis ( Supplementary Fig. 4 ). While the Fluc expression is used as an internal control for the plasmid transfection, it is the chimeric Rluc expression (Rluc-3′UTR or -MREs) that is affected by specific miRNA oligonucleotide mimics (that is, miR-932 mimic). Importantly, we showed the 3′UTR of Act5C is targeted by miR-932 (Ψ-Act5C_3′UTR; Fig. 6a ), whereas the cloned 3′UTRs from Sec61b and His1 did not result in any significant change in expression of the chimeric Rluc (Ψ-Sec61_3UTR and Ψ-His1_3UTR; Fig. 6b,c ). The honeybee-targeting results verify the Drosophila miR-932– Act5C mRNA pull-down interactions and confirm conservation of this mechanism between these insect genera ( Supplementary Fig. 3 ). We similarly used the dual-luciferase system, making plasmid reporter constructs carrying small synthetic sequences of predicted MREs (23 bp plus flanking restriction sites; Supplementary Figs 2 and 4 ). We found the positive-control plasmid constructed using perfectly matched target sites for miR-932 significantly reduced the expression of Rluc in the presence of the miR-932 mimic (Ψ-positive_ctrl; Fig. 6d ), confirming the luciferase reporter system also works with small synthetic oligonucleotides. Of particular importance was the significant downregulation of Rluc carrying the native miR-932 RE in the Act5C 3′UTR (Ψ-Act5C_MRE_wt; Fig. 6e ). This MRE does not have a canonical ‘seed’ (7–8 nt located in the 5′ region of the miRNA) comprising a perfect match with the target site. In this respect the Act5C miR-932 RE is likely to be an atypical ‘seed’ with a 3′-compensatory site [33] . We tested this by introducing mutations in the ‘seed’ and 3′-compensatory regions of the Actin5C MRE showing that the altered sequence disrupts miR-932 targeting of this sequence (Ψ-Act5C_MRE_mut; Fig. 6f ). We also tested whether the antagomir-932 (a-miR-932) inhibits binding of the miR-932 mimic to the cloned target site in the chimeric Rluc gene (Ψ-Act5C_MRE_wt; Supplementary Fig. 5 ). We confirmed that a-miR-932 indeed reduces binding of miR-932 mimic to its target and rescues Rluc expression levels. This effect was not observed with the antagomir scrambled (a-scrambled). Control treatments with antagomirs on their own (a-miR-932 and a-scrambled, respectively) did not result in reduced Rluc expression levels. 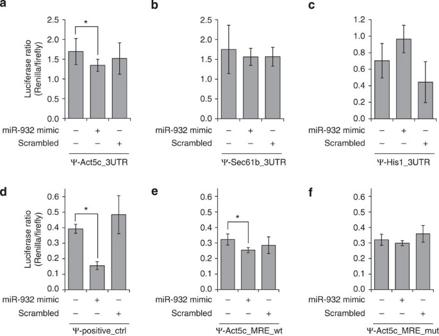Figure 6: Dual-luciferase reporter analysis of miR-932 target interactions. Shown are changes in expression ratio of Firefly (Fluc) and chimericRenillaluciferase (Rluc) containing putative 3′UTR and miRNA regulatory elements (MREs) of target genes treated with and without (±) exogenous miR-932 mimic and scrambled RNA. Welch’s two-samplet-test was used to verify MRE and 3′UTR target associations,t-test*P<0.01. The 3′UTR ofAct5C(a: Ψ-Act5C_3UTR;t=4.35, df=6.55,P<0.01), positive control, perfect match 23-bp miR-932 ‘seed’ sequence (d: Ψ-positive_ctrl;t=6.41, df=5.93,P<0.01) and the native MRE identified in the 3′UTR ofAct5C(e: Ψ-Act5C_MRE_wt;t=5.24, df=3.671,P<0.01) are shown to be significantly downregulated by miR-932. The 3′UTR ofSec61b(b) andHis1(c) were not targeted by the miR-932 mimic. Similarly, the mutant control (f: Ψ-Act5C_MRE_mut) was not downregulated by miR-932. Figure 6: Dual-luciferase reporter analysis of miR-932 target interactions. Shown are changes in expression ratio of Firefly (Fluc) and chimeric Renilla luciferase (Rluc) containing putative 3′UTR and miRNA regulatory elements (MREs) of target genes treated with and without (±) exogenous miR-932 mimic and scrambled RNA. Welch’s two-sample t -test was used to verify MRE and 3′UTR target associations, t-test * P <0.01. The 3′UTR of Act5C ( a : Ψ-Act5C_3UTR; t =4.35, df=6.55, P< 0.01), positive control, perfect match 23-bp miR-932 ‘seed’ sequence ( d : Ψ-positive_ctrl; t =6.41, df=5.93, P< 0.01) and the native MRE identified in the 3′UTR of Act5C ( e : Ψ-Act5C_MRE_wt; t =5.24, df=3.671, P< 0.01) are shown to be significantly downregulated by miR-932. The 3′UTR of Sec61b ( b ) and His1 ( c ) were not targeted by the miR-932 mimic. Similarly, the mutant control ( f : Ψ-Act5C_MRE_mut) was not downregulated by miR-932. Full size image The results of this study highlight how miRNAs and possibly other ncRNAs may regulate the differential expression of protein-coding genes with associative learning (PER-conditioning assay), suggesting that an evolutionary preconfigured molecular system responds to learning and memory of olfactory cues. Our findings are in agreement with recent studies that show there is a general downregulation of protein-coding genes and upregulation of miRNAs associated with learning and memory in honeybees [34] , [35] . These studies report genes involved with cytoskeleton organization, as well as lipid, protein and glucose metabolism are downregulated, and six out of the seven miRNAs reported upregulated in our study after learning were also found upregulated in their work [35] . Although these studies did not test their candidate miRNAs for a functional role in learning and memory, their findings nevertheless substantiate our conclusion that there is a robust preconfigured network of miRNAs that regulate memory formation in bees. When conditioning bees for analysis of differential gene expression, air exposure rather than unpaired conditioning was used as a common control for both odour groups to accommodate direct comparative analysis of gene expression between bees that had been trained to the floral mix and bees trained to the single odour linalool. Using air as a control group means that we cannot completely exclude that simple presentation of the CS (odour, conditioned stimulus) or the US (sugar, unconditioned stimulus) may be involved in the differential expression of some of the coding genes or miRNAs. Nonetheless, when we compare bees trained to single odour (linalool) with bees trained to a floral mix (14 odours) using the PER assay, we see a similar qualitative pattern of molecular regulation compared with the common control irrespective of conditioning treatment ( Supplementary Data 1 ). Linalool is part of the floral mix, and we know that honeybees learn complex scent mixtures based on a reduced number of key odorants [20] , with linalool possibly being one of the key odorants for the mix we used. Hence, floral mix and linalool treatments may indeed elicit a similar qualitative pattern of molecular response in the brain. However, we observed quantitative differences in regulation between the two odour-conditioned groups with floral mix learning eliciting a stronger change in the amount of transcript produced, in particular with respect to miRNA expression ( Fig. 3a ). This increase could be due to more odorants being learnt during conditioning to floral mix [20] compared with the single odour, and the mixture being perceived as a much greater or more concentrated stimulus than linalool alone. Intriguingly, miR-932 had the strongest effect on memory formation in the behavioural assay ( Fig. 5b ) and was not found differentially expressed in the linalool versus air comparison in the qPCR validation ( Fig. 3a ). This is in contrast to the other six miRNAs that were upregulated after linalool conditioning albeit less so than with floral mix conditioning (except for miR-928). Two facts have to be considered when interpreting this result. First, the relative difference of miR-932 expression could be very small due to restricted activation within a confined neural circuit associated with learning a single odorant, and hence not detectable in the qPCR analysis that investigated whole brains. Secondly, miR-932 is embedded and possibly co-regulated with its host gene Nlg2 . The difference in miR-932 up-regulation between mix and single odour treatments may be contingent on the specific (and still unknown) function of Nlg2 in contributing to synapse formation in the whole honeybee brain. Another factor that may have contributed to the variation in miR-932 expression after linalool-conditioning is olfactory receptor plasticity induced by prior experience with linalool [36] . In our study the bees likely had previous memories of linalool considering their immediate response during PER conditioning ( Supplementary Fig. 1 ). Our gene ontology (GO) analysis of DEGs after odour learning showed there was an enrichment of genes involved in metabolic processes, protein localization, regulation of translation and cation homeostasis, including highly conserved molecules such as asparagine synthetase , actin and histone ( Table 1 ; Fig. 1 ). The downregulation of these gene transcripts would clearly affect neurotransmitter profiles, the cytoskeleton and the transcriptional programme of neurons. Asparagine synthetase was the most DEG in odour-conditioned bees ( Fig. 1 ). Considering the essential biosynthetic role of this enzyme (aspartate+glutamine→asparagine+glutamate; Supplementary Fig. 6 ), significant reductions of asparagine synthetase would directly affect the homeostasis of excitatory glutamate and aspartate amino-acid neurotransmitters in the brain [37] that may in turn affect memory acquisition [38] , [39] . Although the neuro-excitatory functions of glutamate interacting with N -methyl- D -aspartic acid (NMDA) receptors found at the post-synaptic membrane have been well studied in both vertebrates and invertebrates, the function of D - and L -aspartic acid and their conversions to NMDA [37] , [40] is less well understood. Importantly, glutamatergic neurons are found in the mushroom bodies of the honeybee brain, and glutamate and NMDA receptors have been shown to play a role in LTM formation in honeybees [41] , [42] , [43] . Thus, our finding that asparagine synthetase is downregulated after olfactory conditioning in bees provides an important addition to current knowledge on the molecular processes regulating learning and memory in this insect model [15] , [27] , [44] . Our network predictions ( Supplementary Data 4 ) show there are >20 miRNAs that potentially interact with asparagine synthetase. Determining the functional significance of asparagine synthetase and its miRNA interactions, controlling levels of excitatory aspartate and glutamate neurotransmitters, will be an important next step in dissecting the molecular underpinnings of olfactory learning and memory. It is intriguing that the majority of differentially expressed coding genes were downregulated after learning in bees. This observation was also made by previous studies using both olfactory [34] and visual [35] learning paradigms in honeybees. Similarly in mammals, there is a pronounced downregulation of gene expression 24 h after long-term-potentiation (LTP) induction, which appears to be partially mediated via time-dependent regulation of miRNA expression [45] . One would have expected that cytoskeletal genes such as actin ( Act5c ) to be upregulated during memory formation [46] . It has been reported that LTM induces synaptic and structural plasticity in the honeybee brain [47] , and several studies show a role for actin in synaptic plasticity, long-term potentiation and memory formation in both insects and vertebrates [46] , [48] , [49] , [50] . We propose that increased levels of miRNAs including miR-932 help to reinforce the persistence of memory by regulating the dynamics of actin polymerization. This hypothesis is supported by evidence from previous studies on appetitive olfactory conditioning in honeybees [49] and aversive olfactory conditioning in Drosophila [51] . The first study showed that inhibition of actin polymerization in the mushroom bodies enhances associative olfactory memory in honeybees [49] , indicating that memory consolidation in insects is facilitated by actin depolymerization, contrary to what is known from mammals [46] . The second study showed that odour-conditioned flies had decreased levels of active G protein Rac (a member of the Rho family of GTPases) suppressing the Rac-based ‘forgetting mechanism’ via activation of cofilin that causes actin depolymerization [51] , [52] . Our hypothesis of miRNA-mediated regulation of actin dynamics during memory formation in honeybees is further supported by vertebrate studies reporting that miRNAs indirectly regulate actin in dendritic spines through Rho and Rac1 GTPase signalling pathways [7] , [53] . We identified over 40 miRNAs that potentially target actin ( Act5C ) in odour-conditioned bees ( Fig. 1 ). We specifically show miR-932 interacts with Drosophila Act5C ( Supplementary Fig. 3 ); and with honeybee Act5C ( Fig. 6a,e,f ), therefore miR-932 would directly affect the actin-related plasticity mechanism involving axon, dendrite and synapse development [7] , [54] , [55] , [56] . We are mindful that combinations of miRNAs including miR-932, miR-210, miR-124 and miR-34 ( Fig. 3 ) probably work together to effectively downregulate Act5C . In this regard, we show the downregulation of miR-932 significantly affects olfactory LTM recall but not memory acquisition ( Fig. 5 ), implying these miRNAs also function in a memory circuit-specific manner. The treatment with a-miR-210 also reduced memory performance compared with the controls, but the difference was only marginal ( Fig. 5 ). This raises the question how miR-210, which has previously been associated with hypoxia response [24] , may affect memory. Considering the extreme sensitivity of neural structures and neurons to hypoxia [57] , we suggest small changes to oxygen levels in metabolic activity neurons may induce expression of miR-210, which in turn targets key molecules including asparagine synthetase and actin . Our study raises questions as to the specific role of these miRNAs in memory consolidation and memory retrieval that will need to be answered. The nested organization of miR-932 and Nlg2 that is putatively involved in synapse development [17] , [18] , [23] is of particular relevance. Aside from finding putative RNA Pol III promoters within 7 kb upstream of miR-932, this intronic miRNA may also be transcribed and processed during Nlg2 expression. The putative co-regulation of Nlg2 with miR-932 and demonstrated interaction with actin and effect on LTM, suggests miR-932 may more directly affect synapse development. However, there is some debate concerning the function of Drosophila Nlg2 (ref. 18 ) and we note the specific role of Nlg2 in the insect brain is yet to be determined. Although there are >10 reported miRNAs known to affect neuronal development, including miR-124, miR132, miR-134, miR-137 and miR-138 that are thought to indirectly regulate actin in dendritic spines of vertebrates through Rho and Rac1 GTPase signalling pathways [7] , [53] , we show miR-932 is the first miRNA described to directly target actin . Interestingly, aside from a documented interaction with CREB1 (refs 10 , 53 ) we predict miR-124 may also interact with insect Actin5c ( Fig. 3b ). We have clearly shown that cholesterol-antisense antagomirs of miR-932 and miR-210 fed to adult bees significantly downregulate these miRNAs in the brain, resulting in observable differences in memory recall in animals that had effectively learnt to associate an odour with a sugar reward ( Fig. 5 ). Cholesterol is an essential component of the nervous system. The concentration of cholesterol is known to be significantly higher in the nervous system than in other tissues, ~25% of the total amount of the cholesterol present in humans is found in the brain [58] where it is locally synthesized. Unlike vertebrates, insects are unable to synthesize cholesterol [59] and until recently, little was known about the mechanisms that regulate the uptake of dietary cholesterol [60] , [61] . Considering the essential dietary requirement for cholesterol in insects and how the brain may be a significant biochemical sink for this lipid, it occurred to us that cholesterol-conjugated RNA antisense technology could be used to functionally analyse miRNAs in the honeybee. The use of cholesterol-antisense RNA technology will help make the honeybee model more tractable for neurobiological research. In summary, there are three principal findings of this study: (1) the PER-associative learning paradigm downregulates protein-coding genes involved in metabolism of neurotransmitters and neuronal remodelling, processes that are likely mediated by increased levels of ncRNAs; (2) miR-932 regulates LTM, but not memory acquisition; (3) miR-932 may contribute to activity-dependent neuronal plasticity by directly targeting actin . These results also raise new questions concerning the molecular response to sensory- and memory stimuli. Aside from miRNAs serving as a dynamic brake on protein synthesis: what signals the release of this brake? Is sensory activity-dependent miRNA interaction multimodal and if so, are the same molecular pathways and processes involved? Our study provides important steps to understand the systems context of miRNA regulation in the brain and puts forward a generalized model how these molecules might contribute to our understanding of higher-order cognitive and sensory processing. Behavioural experiments Foraging honeybees ( Apis mellifera ) were captured at the entrance of an outdoor hive located on campus of the University of Queensland, Brisbane, Australia. Bees were cold-anaesthetized and harnessed in plastic tubes for the proboscis extension response (PER) assay as previously described [20] , [62] . Only bees that were active and extended their proboscis in response to sugar were used. During times when they were not used for behavioural experiments, harnessed bees were fed with 1 M sucrose solution and kept in an incubator in the dark (26 °C, 70% relative humidity). During olfactory learning and LTM formation, honeybees learnt to associate an odour with a sugar reward by blowing an odour for 6 s over the bee’s antennae and 3 s after odour onset presenting a drop of 1 M sucrose solution for 3 s to the bee’s proboscis. Each conditioning trial lasted 6 s with an inter-trial interval (ITI) of 10 min. Odours were delivered using a custom-built olfactometer [20] . Odours were either a mixture of 14 common floral odorants diluted 1:10 in hexane (floral mix, composition and odorant origin as previously described [20] , or linalool diluted 1:10 in hexane (Sigma)). The specific conditioning procedure varied according to experiment, as described below. Microarray sample preparation and hybridization Three groups of 60 honeybees each were conditioned in the PER assay using 12 trials over 2 days, with 6 trials per day (ITI 10 min). This protocol [23] , [36] is used to standardize sensory experience in the experimental bees as much as possible. This is particularly important when using randomly collected bees that differ with respect to prior foraging experience, as brain transcriptome studies show high inter-individual variability that can mask subtle changes in gene expression. Group 1 was conditioned with the floral mix; group 2 with linalool and group 3 were exposed to air serving as a baseline control. Air exposure rather than unpaired conditioning was used as common control for both odour groups to accommodate direct comparison of gene expression between bees that had been trained to the floral mix and bees trained to the single odour linalool. Learning performance over 12 trials was analysed using GLM, which allows testing of binary data. Immediately after the last conditioning trial, bees were killed and their brains dissected, and pooled for each group. Total RNA was extracted from the pooled brains for each group using TRIzol protocol (Invitrogen) combined with column purification (RNeasy Mini Kit, QIAGEN). Complementary DNA (cDNA) synthesis (from 1 μg total RNA), RNA amplification and probe preparation were done with and according to the Amino Allyl MessageAmp II aRNA Amplification Kit (Ambion). Twenty μg of amplified RNA were labelled with Cy3 or Cy5 dye (RPN5661, GE Healthcare). Probe purification was done using the MinElute PCR Purification Kit (QIAGEN). Microarray data have been deposited in the Gene Expression Omnibus (GEO accession number GSE51795). We followed the same experimental procedures as previously described [63] . Pairs of RNA samples were labelled with Cy3 or Cy5 fluorophores and hybridized to the same slide following the experimental design: (1) linalool versus air; (2) floral mix versus air. Dye swaps were done for each comparison. Computational analysis of microarray data The microarray slides were scanned using an Axon Genepix 4000B scanner (Molecular Devices) with GenePix Pro 6.0 software (Agilent Technologies, Santa Clara, CA) at a 10-micron resolution, during which Cy3 was excited with a green laser (532 nm) and Cy5 with a red laser (635 nm). For image quantification, we used GenePix Pro 6.0 software with default parameters. For analysis, all normalizations and fold-change calculations were performed using the functions in the library Limma of the R/Bioconductor package [64] as previously described [63] . A gene was considered differentially expressed when the adjusted P value (using Bonferroni correction) was <0.05. Gene annotation of DEGs All probes found to be differentially expressed from the microarray analysis were identified using the BeeBase Official Gene Set version 3.2 ( http://hymenopteragenome.org/beebase/ ) [65] and with GenBank at the National Center for Biotechnology Information (NCBI; http://www.ncbi.nlm.nih.gov/ ). All DEGs were annotated according to GO terms for Biological Process based in the Drosophila melanogaster orthologous sequences. Validation of microarray results by qRT-PCR The same RNA samples were used for qRT-PCR to validate microarray results. First-strand cDNA was synthesized by reverse transcription using 1 μg of total RNA, SuperScript II reverse transcriptase and oligo dT primer (Invitrogen). We designed specific primers for 23 genes differentially expressed from the microarray analysis ( Supplementary Table 1 ). The ribosomal protein L8 ( RPL8 ) gene was used as an endogenous control and the air sample was used as a calibrator for the quantitative analysis. The real-time quantitative RT-PCR assays were performed in a LightCycler 480 (Roche). Amplifications were carried out in 20-μl reaction volumes, containing 10 μl SYBR Green Master Mix 2 × (Applied Biosystems), 1 μl first-stranded cDNA, 7.4 μl water and 1 pmol of each gene-specific primer. PCR conditions were 50 °C for 2 min and 95 °C for 10 min, followed by 40 cycles of 95 °C for 15 s and 60 °C for 1 min. To check reproducibility, each SYBR green assay was performed in triplicate. PCR efficiency values ( E ) were calculated for each gene from the given slope after running standard curves and following the formula E =10(−1/Slope). The relative transcripts levels were calculated using the 2 −ΔΔCT method. Analysis of PPI network We used PPI data available in the BioGRID database (version 3.2.101) [21] for the fruit fly D. melanogaster predictions. To build the PPI network for the honeybee genes, we first identified all putative orthologous genes between fruit fly and honeybee using the ‘reciprocal best hit’ method [66] ( Supplementary Data 7 ). The PPI network is constructed by connecting all first-degree-interacting protein neighbours of the DEGs. Network visualization and functional analysis was performed using Cytoscape [67] . We used ClueGO cytoscape plugin [68] to find GO categories statistically enriched in the PPI network. The P value was calculated using the Fisher exact test and adjusted using Benjamini–Hochberg correction. We tested the statistical significance of the connections between the DEGs for the PPI network. The method involves creating networks from 100 genes sampled from the DEGs and from the whole genome (control). We measured three basic properties: (1) average degree, (2) average path length and (3) density of the network, and checked whether the distribution of those structural properties were the same in the DEG PPI networks and in the random networks. We used the non-parametric Kolmogorov–Smirnov test to test the hypothesis of random connections among DEGs. Computational analysis of the miRNA-target network To construct the miRNA-target network for the downregulated genes, we used only those A. mellifera miRNAs found in the miFam (miRNA family) feature available in the miRbase database (v. 20), which provides family classification information of homologous miRNA hairpin sequences. miRNA-target predictions were performed using the RNAhybrid programme [69] . The database of putative 3′UTR sequences was created by retrieving 1,000 nt sequence downstream of the stop codon for orthologous genes of A. mellifera and D. melanogaster . The network of miRNAs and their respective target genes was created by identifying the presence of at least one predicted target site with free energy ≤−20. We used Cytoscape [67] to visualize, compare and construct the composite miRNA and PPI network conserved in honeybee and fruit fly. Expression patterns of relevant miRNAs identified from the putative miRNA-target network were validated by qRT-PCR analysis using the same RNA samples as used for the microarray study ( Supplementary Table 2 ). The 18S rRNA gene was used as endogenous control; the PCR assay was performed as a technical triplicate to check reproducibility, and calculation methods were performed as described above. In situ hybridization of candidate miRNA Forager honeybee brains were stained as previously described [17] . Whole-brain sections were hybridized with the LNA miR-210 and miR-932 probes (Exiqon) and with a negative control (LNA scrambled sequence). Probe mix (150 μl) (1.0 μg ml −1 ) was added per section and denatured at 95 °C. Hybridization was carried out at 55 °C overnight. Sections were rinsed and treated with 10 μg ml −1 RNaseA (Qiagen: #19101) for 30 min at 37 °C and washed using PBS and reducing concentrations of SSC and SSC+0.1% SDS. The slides were rinsed in wash buffer 1, and treated with 2% blocking solution (4 g blocking reagent (Roche: # 11 096 176 001) for 30 min at room temperature (RT). Each section was incubated with 150 μl alkaline phosphatase-labelled anti-DIG antibody (Roche: #11 093 274 910) at 1:500 in blocking buffer for at least 2 h at RT or overnight at 4 °C. To reduce nonspecific binding, slides were washed in wash buffer 1 and then in wash buffer 2. Each section was then covered with 200 μl of freshly prepared colour solution (wash buffer 2 with 200 μl of a nitroblue tetrazolium chloride (NBT)/(BCIP) mix from Roche: #11 681 451 001), and 10 μl of 1 M Levamisole (Sigma: # L9756) final concentration of 1 mM). Colour development appeared within 30 min to 1 h at RT. The reaction was stopped by rinsing in wash buffer 3 and with deionized water. Nonspecific staining was further removed by using a series of ethanol washes; slides were mounted and sealed with glass cover slips. Images were captured using bright-field illumination microscopy. Computational analysis of miRNA promoter regions The upstream regions of miR-932 and miR-210 were retrieved from the honeybee genome sequence version 4.5 (Amel 4.5; http://hymenopteragenome.org/beebase/ ) [65] . The RNA Pol III REs were represented as a position-specific scoring matrix based on the consensus A-box (5′-TRGCNNARYNGG-3′) and B-box (5′-GGTTCRANNCC-3′) sequences [31] using TAMO python module [70] . The identification of A/B boxes with at least 60% of similarity to the consensus sequences was performed using TAMO python module. Functional validation of miRNAs Four groups of 20 bees each were harnessed as described above, and treated with specifically designed antisense miRNA sequences (antagomir-932, antagomir-210 and scrambled ‘nonsense’ sequence) conjugated with a cholesterol moiety (Exiqon). Harnessed bees were fed with 1 μg antagomir diluted in 1 μl sugar solution. Group one was fed only sugar (behavioural control), group two was fed ‘scrambled’ (molecular control), group three received a-miR-932 and group four received a-miR-210. Twenty-four hours after treatment, bees were conditioned in the PER assay using six learning trials (ITI 10 min) with linalool 1:10 as the conditioning odour. Twenty-four hours after conditioning (that is, 48 h after treatment), they were tested for LTM recall in the PER assay. Only bees that consistently showed proboscis extension in response to sugar during the entire 48 h were used for analysis. The experiment was replicated until at least 30 individuals per group were trained and tested. Learning performance over six trials as well as memory recall was analysed using GLM with automatic correction for multiple comparisons, and trial and treatment as factors. GLM allows testing of binary data. To validate the efficiency of the non-invasive miRNA inhibition method, four further groups of 20 bees each were treated as above with a-miR-932, a-miR-210, scrambled and sugar, but without olfactory conditioning. Twenty-four and 48 h after treatment, their brains were dissected, and expression of miR-932 and miR-210 was quantified using qRT-PCR with the sugar group as a calibrator for ΔΔCT, and scrambled as a treatment control (baseline). The housekeeping gene 18S rRNA was used as an endogenous control. We extracted total RNA from five brains per sample of each treatment and with three biological replicate experiments for qRT-PCR analysis. To estimate the relative miRNA expression (miRNA–sugar/scrambled–sugar), we averaged all three biological replicates and used the ΔΔCT method. Validation of miRNA-target genes by the pull-down assay Approximately 7 × 10 6 Drosophila S2 cells were collected and centrifuged (1,000 g , 3 min, RT). The supernatant media was removed and the cells were resuspended in 500 μl cell lysis buffer, the tubes were left on ice for 5 min and centrifuged (9,000 g ) for 10 min at RT. The cytoplasmic lysate was transferred to new tubes and either bi-miR-932 or bi-scr (Exiqon) was added in the final concentration 2 pmol μl −1 . The cytoplasmic lysate and bi-miRNA solution was incubated at 75 °C for 3 min, left at RT for 5 min and incubated for 37 °C for 60 min. For the control condition, total RNA was extracted from S2 cells cytoplasmic lysate before being complexed with miRNA mimic solution and the Dynabeads M-280 Streptavidin (Invitrogen) were washed and prepared according to the manufacturer’s protocol (Invitrogen). For each treatment (miR-932 and scrambled mimic), 500 μl of Dynabeads was used. The cytoplasmic lysate and bi-miRNA solution was added to the Dynabeads and incubated for 1 h at 10 r.p.m. at RT (Intelli Mixer ELMI). After incubation, the supernatant was removed and the Dynabeads were washed three times with 500 μl lysis buffer. miRNA–mRNA complexes were released from the Dynabeads by adding 500 μl Tris-HCl (10 mM, pH 7.5) and incubation at 80 °C for 5 min followed by 5 min at RT. Total RNA was extracted as per the TRIzol (Invitrogen) method and used as a template to measure transcript levels with qRT-PCR ( Supplementary Table 3 ). miRNA-target validation using the luciferase reporter system We designed primers flanking the binding-site regions in the 3′UTR of Act5C , Sec61b and His1 genes ( Supplementary Table 4 ). XhoI and NotI restriction sites were added to the 5′ end of the forward and reverse primers, respectively. The designed primers were used to amplify the 3′UTRs from bee brain cDNA. In addition, we designed forward and reverse oligonucleotides to be used as control sequences (containing one perfect match for the entire miR-932 sequence) and small synthetic MREs (containing the putative miR-932-binding site) ( Supplementary Table 5 ). Both synthetic sequences contain the restriction sites for NotI and XhoI and were annealed in an annealing buffer (100 mM Tris-Hcl pH 7.5, 1 M NaCl, 10 M EDTA) for 40 min at 90 °C, followed by 2 h at RT. psiCHECK2 vector (2 μg) and the amplified 3′UTR or the synthetic MRE (700 ng) were NotI and XhoI digested and isolated fragment ligated with 50 ng of appropriately RE-cut dephosphorylated psiCHECK2 vector. COS-7 cells (5 × 10 4 cells per well) were co-transfected for 24 h with psiCHECK2 (containing or not the candidates 3′ UTR) (Promega, 200 ng per well), miRIDIAN mimic miR-932 or scrambled sequence (Dharmacon, 40 pmol per well) using Lipofectamine LTX with Plus Reagent (Invitrogen, 3 μl per well) according to the manufacturer’s instruction. Dual-Luciferase Reporter Assay System (Promega) was used to determine Firefly and Renilla luciferase activities. We also examined the blocking effect of 60 pmol of cholesterol-conjugated antagomirs (a-miR-932 and control a-scrambled) to verify binding of miR-932 mimic with the Act5c regulatory site. The expression of Renilla luciferase (Rluc) was measured using the same protocol as described above ( Supplementary Fig. 5 ). Statistical analysis Statistical analysis was conducted as indicated in the text, figure legends and online methods using R. Where required P values were adjusted using Bonferroni or Benjamini–Hochberg correction. All t -tests used were two sided, and appropriate tests were applied depending on whether data met assumptions of equal sample size and variance. Accession codes: Microarray data have been deposited in the Gene Expression Omnibus under GEO accession code GSE51795 . How to cite this article: Cristino, A. S. et al. Neuroligin-associated microRNA-932 targets actin and regulates memory in the honeybee. Nat. Commun. 5:5529 doi: 10.1038/ncomms6529 (2014).